Spin-orbital entangled molecularjeffstates in lacunar spinel compounds The entanglement of the spin and orbital degrees of freedom through the spin-orbit coupling has been actively studied in condensed matter physics. In several iridium oxide systems, the spin-orbital entangled state, identified by the effective angular momentum j eff , can host novel quantum phases. Here we show that a series of lacunar spinel compounds, GaM 4 X 8 (M=Nb, Mo, Ta and W and X=S, Se and Te), gives rise to a molecular j eff state as a new spin-orbital composite on which the low-energy effective Hamiltonian is based. A wide range of electron correlations is accessible by tuning the bandwidth under external and/or chemical pressure, enabling us to investigate the cooperation between spin-orbit coupling and electron correlations. As illustrative examples, a two-dimensional topological insulating phase and an anisotropic spin Hamiltonian are investigated in the weak and strong coupling regimes, respectively. Our finding can provide an ideal platform for exploring j eff physics and the resulting emergent phenomena. Spin-orbit coupling (SOC) is a manifestation of Einstein’s theory of relativity in condensed matter systems. Recently, SOC has attracted a great deal of attention since it is a main ingredient for spintronics applications [1] , [2] , induces novel quantum phases [3] , [4] and generates new particles and elementary excitations [5] , [6] . Moreover, when incorporated with electron correlations, SOC can give rise to even more fascinating phenomena [7] , [8] . In the iridium oxide family, where the IrO 6 octahedron is the essential building block, various quantum phases have been predicted or verified according to the electron correlation strength on top of the large SOC of the Ir 5 d t 2g orbital: topological band insulator for weak coupling [9] , [10] , Weyl semi-metal, axion insulator, non-Fermi liquid and TI* phases for intermediate coupling [11] , [12] , [13] , [14] , [15] , and topological Mott insulator and quantum spin liquid phases for strong coupling [7] , [16] , [17] . Emergence of the spin-orbital entangled j eff states induced by SOC [18] , [19] is the key feature to host all the above phases, yet the existence of such states is limited to a small number of iridate compounds only. Here, the series of lacunar spinel compounds [20] , [21] , GaM 4 X 8 , where early 4 d or 5 d transition metal atoms occupy the M-site, are found to provide the molecular form of the j eff basis in their low-energy electronic structures. The idealness of the molecular j eff state is guaranteed by the formation of the M 4 metal cluster and the large SOC. Combined with the ability to control the electron correlation from the weak to strong coupling limit, the lacunar spinels can manifest themselves as the best candidates to demonstrate this so-called j eff physics. Formation of the molecular j eff states in GaTa 4 Se 8 The chemical formula and crystal structure of the GaM 4 X 8 lacunar spinels are easily deduced from the spinel with half-deficient Ga atoms, that is, Ga 0.5 M 2 X 4 . Due to the half removal of the Ga atoms, the transition metal atoms are strongly distorted into the tetrahedral center as denoted by the red arrows in Fig. 1a , and a tetramerized M 4 cluster appears. The M 4 cluster yields a short intra-cluster M–M distance, naturally inducing the molecular states residing on the cluster as basic building blocks for the low-energy electronic structure. On the other hand, the large inter-cluster distance results in a weak inter-cluster bonding and a narrow bandwidth of the molecular states. 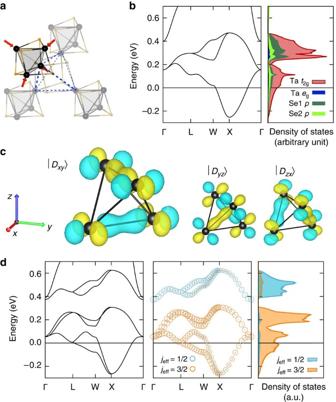Figure 1: Molecular form of spin-orbital entangledjeffstates in GaTa4Se8. (a) The connectivity between the neighbouring M4clusters and the local distortion of each cluster. (b) Band structure and PDOS of GaTa4Se8without SOC. (c) Three Wannier orbitals constructed from the triplet molecular orbital bands near the Fermi level. (d) Band structure and DOS with SOC, projected onto thejeff=1/2 and 3/2 subspaces. The size of the circle in the band structure shows the weight of each subspace in each Bloch state. Figure 1: Molecular form of spin-orbital entangled j eff states in GaTa 4 Se 8 . ( a ) The connectivity between the neighbouring M 4 clusters and the local distortion of each cluster. ( b ) Band structure and PDOS of GaTa 4 Se 8 without SOC. ( c ) Three Wannier orbitals constructed from the triplet molecular orbital bands near the Fermi level. ( d ) Band structure and DOS with SOC, projected onto the j eff =1/2 and 3/2 subspaces. The size of the circle in the band structure shows the weight of each subspace in each Bloch state. Full size image As a representative example of the lacunar spinels, we investigate the electronic structure of GaTa 4 Se 8 ( Fig. 1b–d ). Figure 1b shows the band structure and the projected density of states (PDOS) of GaTa 4 Se 8 in the absence of SOC. In consistency with previous studies [21] , [22] , [23] , the triply degenerate molecular t 2 bands occupied by one electron are located near the Fermi level with a small bandwidth of ~0.75 eV. As shown in the PDOS plot, the molecular t 2 bands are dominated by Ta t 2g orbital components; the small admixture of Se 5 p and the strong tetramerization imply that the molecular t 2 states consist of direct bonding between Ta t 2g states. The molecular nature of the low-energy electronic structure can be visualized by adopting the maximally localized Wannier function scheme [24] , [25] . The three molecular t 2 Wannier functions depicted in Fig. 1c read where D α and d α denote the molecular t 2 and atomic t 2g states, respectively, and i is a site index indicating the four corners of the M 4 cluster. Each D α originates from a σ -type strong bonding between the constituent t 2g orbitals in the M 4 cluster. (See Supplementary Note 1 , Supplementary Fig. 1 and Supplementary Table 1 for details on the molecular t 2 Hamiltonian.) Owing to the exact correspondence between the molecular t 2 and the atomic t 2g states, as revealed in equation 1, the molecular t 2 triplet carries the same effective orbital angular momentum l eff =1 as the atomic t 2g orbital [18] . By virtue of SOC, the l eff =1 states are entangled with the s =1/2 spin, and two multiplets designated by the effective total angular momentum j eff =1/2 and 3/2 emerge. The band structure and PDOS of GaTa 4 Se 8 in the presence of SOC verify the above j eff picture ( Fig. 1d ); the molecular t 2 bands split into upper j eff =1/2 and lower j eff =3/2 bands. The separation between the two j eff subbands is almost perfect owing to the large SOC of the Ta atoms as well as the small bandwidth of the molecular t 2 band. An alternative confirmation of the j eff picture can also be given by constructing the Wannier function from each of the j eff subbands, which shows a 99% agreement with the ideal molecular j eff states. (See Supplementary Fig. 2 .) Consequently, the electronic structure of GaTa 4 Se 8 can be labelled as a quarter-filled j eff =3/2 system on a face-centered cubic lattice. Robust j eff -ness in the GaM 4 X 8 series The aforementioned j eff -ness in GaTa 4 Se 8 remains robust in the GaM 4 X 8 series with a neighbouring 5 d transition metal (M=W) as well as the 4 d counterparts (M=Nb and Mo). Among the series, M=W compounds have not been reported previously in experiments; thus we use optimized lattice parameters by structural relaxations. In Fig. 2a–d , the electronic structures of GaTa 4 Se 4 Te 4 [26] , GaW 4 Se 4 Te 4 , GaNb 4 Se 8 [21] and GaMo 4 Se 8 [27] are shown—band structure, PDOS and Fermi surface with projection onto the molecular j eff states. In Fig. 2a,b , one can see the clear separation and identification of the higher j eff =1/2 doublet and the lower j eff =3/2 quartet driven by the large SOC of the 5 d transition metal atoms. The overall band dispersions are quite similar, except for the location of the Fermi level; the M=Ta and M=W lacunar spinels are well characterized by the quarter-filled j eff =3/2 and the half-filled j eff =1/2 systems, respectively. In 4 d compounds, the separation between the j eff subbands is reduced due to the smaller SOC compared with that of the 5 d systems ( Fig. 2c,d ). Nevertheless, there is a discernible splitting between the j eff =1/2 and 3/2 bands, which is comparable to or even better than that in the prototype j eff compounds, Sr 2 IrO 4 and Ba 2 IrO 4 [28] . 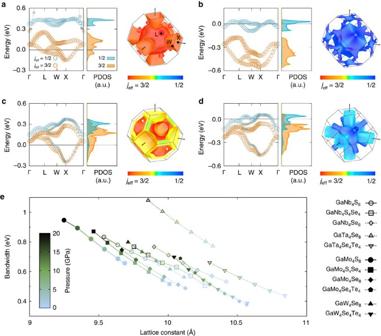Figure 2:jeff-ness in the GaM4X8series. The molecularjeff-projected band structures, DOS and the Fermi surfaces of (a) GaTa4Se4Te4, (b) GaW4Se4Te4, (c) GaNb4Se8and (d) GaMo4Se8are presented. (e) The relation between the external hydrostatic pressure, lattice constant and bandwidth of the moleculart2bands in the absence of SOC. Figure 2: j eff -ness in the GaM 4 X 8 series. The molecular j eff -projected band structures, DOS and the Fermi surfaces of ( a ) GaTa 4 Se 4 Te 4 , ( b ) GaW 4 Se 4 Te 4 , ( c ) GaNb 4 Se 8 and ( d ) GaMo 4 Se 8 are presented. ( e ) The relation between the external hydrostatic pressure, lattice constant and bandwidth of the molecular t 2 bands in the absence of SOC. Full size image To acquire a well-identified j eff band, we need the j eff state as a local basis, and the inter-orbital hopping terms between the j eff subspaces should be suppressed. Hence, there are three important conditions to realize the ideal j eff system: high symmetry protecting the l eff =1 threefold orbital degeneracy, small bandwidth minimizing the inter-orbital mixing and large SOC fully entangling the spin and orbital degrees of freedom. The lacunar spinel compounds comfortably satisfy the above conditions; the tetrahedral symmetry of the M 4 cluster protects the orbital degeneracy, the long inter-cluster distance leads to the small bandwidth and a large SOC is inherent in 4 d and 5 d transition metal atoms. Figure 2e introduces one important controlling parameter—the bandwidth. By changing the inter-cluster distance via external pressure and/or by substituting chalcogen atoms, the bandwidth of the molecular t 2 band can be tuned over a wide range. In the M=Ta series, for example, the bandwidth varies from 0.4 to 1.1 eV. Consequently, the effective electron correlation strength, given by the ratio between the bandwidth and the on-site Coulomb interactions, can be controlled to reach from the weak to the strong coupling regime. In fact, the bandwidth-controlled insulator-to-metal transitions were observed in GaTa 4 Se 4 and GaNb 4 Se 4 [23] , [29] , implying that both the weakly and strongly interacting limits are accessible in a single compound. Effective Hamiltonian From the apparent separation between the j eff subbands, as well as the similar band dispersions, the GaM 4 X 8 series are governed by a common effective Hamiltonian composed of two independent j eff =1/2 and 3/2 subspaces, that is, . (See Supplementary Notes 2 and 3 .) Therefore, the compounds with M=Nb/Ta and M=Mo/W are described by the quarter-filled and the half-filled systems, respectively. The nearest-neighbor hopping terms for each subspace are written as where S 1/2 and S 3/2 are the j eff =1/2 and 3/2 pseudospin matrices, respectively, and Γ are the 5-component Dirac Gamma matrices. t 0 and t Q ’s are even, and t D ’s are odd functions under the spatial inversion; t D ’s are allowed by the inversion asymmetry of the M 4 cluster. The pseudospin-dependent hopping terms t D and t Q can be interpreted as the effective magnetic dipolar and quadrupolar fields acting on the hopping electron, respectively. DFT+SOC+ U calculations So far, we have discussed about the j eff -ness without containing electron correlations, which provides a valid picture in the weak coupling regime. Once taking electron correlations into account, one important question arises on the robustness of the molecular j eff states under the influence of the on-site Coulomb interaction. To answer this question, we perform DFT+SOC+ U calculations for GaTa 4 Se 4 Te 4 , GaW 4 Se 4 Te 4 , GaNb 4 Se 8 and GaMo 4 Se 8 . We consider two simplest magnetic configurations, ferromagnetic and antiferromagnetic order, and the antiferromagnetic solutions for each compound are shown in Fig. 3 . In the 5 d compounds, the molecular j eff states remain robust with developing a SOC-assisted Mott gap within each j eff subspace ( Fig. 3a,b ). For the 4 d compounds, the j eff character is enhanced from the non-interacting cases in Fig. 2c,d ; the occupied states in GaNb 4 Se 8 ( Fig. 3c ) and the unoccupied states in GaMo 4 Se 8 ( Fig. 3d ) are dominated by j eff =3/2 and 1/2 characters, respectively. The strengthened j eff character by the cooperation with electron correlations is consistent with the recent theoretical results on Sr 2 IrO 4 [28] , [30] . See the Supplementary Note 4 , Supplementary Figs 3–6 and Supplementary Tables 2–5 for more details. 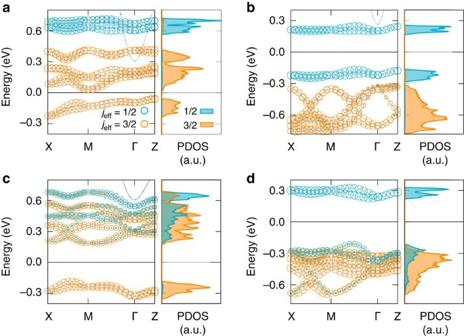Figure 3: DFT+SOC+Ucalculations. Thejeff-projected band structure and DOS of (a) GaTa4Se4Te4, (b) GaW4Se4Te4, (c) GaNb4Se8and (d) GaMo4Se8with the presence of electron correlations and antiferromagnetic order. Figure 3: DFT+SOC+ U calculations. The j eff -projected band structure and DOS of ( a ) GaTa 4 Se 4 Te 4 , ( b ) GaW 4 Se 4 Te 4 , ( c ) GaNb 4 Se 8 and ( d ) GaMo 4 Se 8 with the presence of electron correlations and antiferromagnetic order. Full size image The effective Hamiltonian of the lacunar spinel series has intriguing implications both in the weak and strong coupling regimes. As suggested in previous studies [3] , [9] , [31] , the effective fields exerted on the hopping electron can induce a topological insulating phase in the weak coupling regime. In fact, a non-trivial band topology is realized within the molecular j eff bands in-thin film geometries: the monolayer ( Fig. 4a ) and the bilayer thin film ( Fig. 4b ) of the M 4 clusters normal to the (111) direction. Each system corresponds to the triangular and honeycomb lattice, respectively, and the inter-layer coupling enhanced by a factor of three is adopted in the bilayer system. Non-trivial gaps emerge in the half-filled j eff =3/2 bands in the monolayer and the half-filled j eff =1/2 bands in the bilayer system. A two-dimensional (2D) topological insulator phase is indicated by an odd number of edge Dirac cones at time-reversal invariant momenta in ribbon geometries ( Fig. 4a,b ). Such 2D geometries might be feasible with the help of the state-of-the-art epitaxial technique prevailing in oxide perovskite compounds [32] , or by mechanically cleaving the single crystal to get clean surfaces as done in previous studies on GaTa 4 Se 8 [33] , [34] . 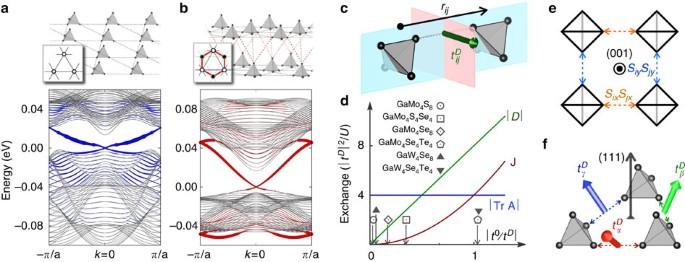Figure 4: Topological insulating phases and anisotropic spin model. The one-dimensional band structure of (a) half-filledjeff=3/2 monolayer and (b) half-filledjeff=1/2 bilayer M4ribbons (20 unit cell width). The insets show schematic top view of each system, where the thin grey and the thick red lines represent the intra- and the inter-planar bonding, respectively. The thickness of the coloured fat lines in the band structure represent the weights on the edge. (c) Two mirror planes (blue and red) existing in between the neighbouring M4clusters determine the direction ofillustrated as green arrow. (d) Magnitudes of Heisenberg (dark red), Dzyaloshinskii–Moriya (green) and pseudodipolar (blue) exchange interactions as a function of |t0/tD|. The magnitude of |t0/tD| for each of the M=Mo/W compounds is marked on the horizontal axis. (e) The 90°- and (f) the 60°-compass interactions are realized on (001) and (111) M4monolayers, respectively. Figure 4: Topological insulating phases and anisotropic spin model. The one-dimensional band structure of ( a ) half-filled j eff =3/2 monolayer and ( b ) half-filled j eff =1/2 bilayer M 4 ribbons (20 unit cell width). The insets show schematic top view of each system, where the thin grey and the thick red lines represent the intra- and the inter-planar bonding, respectively. The thickness of the coloured fat lines in the band structure represent the weights on the edge. ( c ) Two mirror planes (blue and red) existing in between the neighbouring M 4 clusters determine the direction of illustrated as green arrow. ( d ) Magnitudes of Heisenberg (dark red), Dzyaloshinskii–Moriya (green) and pseudodipolar (blue) exchange interactions as a function of | t 0 / t D |. The magnitude of | t 0 / t D | for each of the M=Mo/W compounds is marked on the horizontal axis. ( e ) The 90°- and ( f ) the 60°-compass interactions are realized on (001) and (111) M 4 monolayers, respectively. Full size image In the strong coupling regime, the large on-site Coulomb terms are added to the kinetic Hamiltonian, and the hopping terms are treated as perturbations. The localized j eff pseudospins become low-energy degrees of freedom and exchange interactions between the neighbouring j eff moments emerge. In the simplest example, the one-band Hubbard model within the half-filled , the resulting spin Hamiltonian for the j eff =1/2 moments is written as [35] , [36] among the exchange interaction terms, the Dzyaloshinskii–Moriya D ij and the pseudodipolar interaction A ij depend on , whose direction is determined by the two mirror planes, as illustrated in Fig. 4c (details in Supplementary Note 5 ). As shown in Fig. 4d , the relative magnitude of each exchange term is changed with different chalcogen atoms, so that systematic study of the anisotropic Hamiltonian in equation 3 can be made in the M=Mo/W compounds. Especially, GaMo 4 S 8 and GaW 4 Se 8 satisfies the limit of | t 0 / t D |→0, where the spin Hamiltonian becomes highly anisotropic and bond direction dependent such that with . In addition to the Heisenberg term, the Hamiltonian contains the bond-dependent and Ising-like pseudodipolar interaction, called as a Heisenberg-compass model [37] . It can be further reduced to distinct 2D spin models in thin-film geometries. Figure 4e,f shows two examples—the (001) and (111) monolayer lead to the 90°- and 60°-compass model with the Heisenberg exchange term on a square and a triangular lattice, respectively. The j eff =3/2 systems in the strong coupling limit could also have a significant implication in terms of unconventional multipolar orders [38] , [39] , [40] . On top of the nonmagnetic insulating behaviour, the weak tetragonal superstructure and the anomalous magnetic response observed in GaNb 4 S 8 at T~31 K [41] could give some clues on the quadrupolar ordered phase as well as the spin liquid phase suggested in ref. 39 , which promptly calls for further research on the j eff =3/2 spin model. The formation of the M 4 cluster and SOC are the essential requisites to realize the molecular j eff state in these 3D intermetallic compounds. The strong tetramerization sustains the isolated molecular bands with threefold orbital degeneracy and narrow bandwidth, and the large SOC fully entangles the spin and orbital components. The existence of the pure quantum state has been shedding light on studying the ideal quantum model systems in strongly correlated physics; the Hubbard Hamiltonian or the frustrated spin Hamiltonian based on the pure spin-half state has been realized in several organic compounds [42] , [43] , [44] . Likewise, the molecular form of the ideal j eff state as a pure quantum state might be of great use to explore the emergent phenomena in the spin-orbit-coupled correlated electron systems. First-principles calculations Structural optimizations were done with the projector augmented wave potentials and the PBEsol [45] generalized gradient approximation as implemented in the Vienna ab initio Simulation Package [46] , [47] . Momentum space integrations were performed on a 12 × 12 × 12 Monkhorst-Pack grid, and a 300-eV energy cutoff was used for the plane-wave basis set. The force criterion was 10 −3 eV Å −1 , and the pressures exerted were estimated by using the Birch–Murnaghan fit. For the electronic structure calculations, we used OPENMX code [48] based on the linear-combination-of-pseudo-atomic-orbital basis formalism. Four hundred Rydberg units of energy cutoff was used for the real-space integration. SOC was treated via a fully relativistic j -dependent pseudopotential in a non-collinear scheme. Simplified DFT+ U formalism by Dudarev et al . [49] , implemented in OPENMX code [50] , was adopted in the DFT+SOC+ U calculations. U eff ≡ U − J =2.5 and 2.0 eV was used for the 4 d and 5 d compounds, respectively. How to cite this article: Kim, H.-S. et al . Spin-orbital entangled molecular j eff states in lacunar spinel compounds. Nat. Commun. 5:3988 doi: 10.1038/ncomms4988 (2014).